Total synthesis of atropurpuran Due to their architectural intricacy and biological significance, the synthesis of polycyclic diterpenes and their biogenetically related alkaloids have been the subject of considerable interest over the last few decades, with progress including the impressive synthesis of several elusive targets. Despite tremendous efforts, conquering the unique structural types of this large natural product family remains a long-term challenge. The arcutane diterpenes and related alkaloids, bearing a congested tetracyclo[5.3.3.0 4,9 .0 4,12 ]tridecane unit, are included in these unsolved enigmas. Here we report a concise approach to the construction of the core structure of these molecules and the first total synthesis of (±)-atropurpuran. Pivotal features of the synthesis include an oxidative dearomatization/intramolecular Diels-Alder cycloaddition cascade, sequential aldol and ketyl-olefin cyclizations to assemble the highly caged framework, and a chemoselective and stereoselective reduction to install the requisite allylic hydroxyl group in the target molecule. Three-dimensionally complex and highly cage-like molecules represent some of the amazing natural products that provide both enormous benefits and new challenges to mankind [1] . For instance, the polycyclic diterpenes and their alkaloidal congeners, both featuring difficult chemical structures and possible medicinal applications, fall into such a category [2] , [3] , [4] . From a biogenetic viewpoint, the formation of structurally diverse diterpenes relies on cyclization and oxidation stages, starting from geranylgeranyl diphosphate [5] , [6] , and the introduction of nitrogen atoms into the well-established diterpene skeletons affords the diterpenoid alkaloids [7] , [8] . While the genera of Aconitum and Delphinium provided rich sources for various types of these pseudo-alkaloids [7] , only a few of their parent diterpene molecules were isolated from nature. As illustrated in Fig. 1a , identification of the atisane-, hetidane- and arcutane-type diterpenes ( 1 – 3 , Fig. 1a ) belonged to such exceptional cases [9] , [10] , [11] in which the corresponding natural alkaloids ( 4 – 6 ) were isolated [12] , [13] , [14] , [15] , [16] . All these structural types were biosynthetically derived from atisane diterpenes and are closely related to each other. Specifically, based on the atisane/atisine cores, C14–C20 bond construction afforded hetidanes/hetidines [17] and further bond rearrangement (C10–C20→C5–C20) gave rise to the arcutane/arcutine frameworks [17] , [18] . 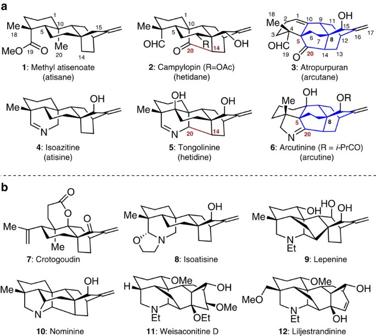Figure 1: Three-dimensionally cage-like diterpenes and diterpenoid alkaloids. (a) Selected members of three related types of diterpenes and their alkaloidal congeners. Among them, the arcutane diterpenes (that is,3) and arcutine alkaloids (that is,6), containing a unique tetracyclo[5.3.3.04,9.04,12]tridecane moiety (shown in blue bonds) and two all-carbon bridgehead quaternary centres (C5 and C8), posed formidable synthetic challenges. (b) Recent accomplishments in the total synthesis of complex atisane-type diterpenes and diterpenoid alkaloids. Ac, acetyl;i-Pr, isopropyl. Figure 1: Three-dimensionally cage-like diterpenes and diterpenoid alkaloids. ( a ) Selected members of three related types of diterpenes and their alkaloidal congeners. Among them, the arcutane diterpenes (that is, 3 ) and arcutine alkaloids (that is, 6 ), containing a unique tetracyclo[5.3.3.0 4,9 .0 4,12 ]tridecane moiety (shown in blue bonds) and two all-carbon bridgehead quaternary centres (C5 and C8), posed formidable synthetic challenges. ( b ) Recent accomplishments in the total synthesis of complex atisane-type diterpenes and diterpenoid alkaloids. Ac, acetyl; i -Pr, isopropyl. Full size image Over the past decade, the synthetic community has made great efforts in pursuit of the total synthesis of atisane diterpenes and their related diterpenoid alkaloids with some notable successes [2] , [3] , [4] , [19] , [20] , [21] , [22] , [23] , [24] , [25] , [26] , [27] , [28] . The teams of Carreira and Liu reported creative solutions for the total synthesis of a 3,4-seco atisane diterpene (crotogoudin, 7 , Fig. 1b ) [23] , [26] , respectively. Baran and co-workers disclosed a unified access to methyl atisenoate ( 1 ), isoatisine ( 8 ) and the hetidine skeleton from a common intermediate [24] . Additionally, the Fukuyama group contributed to the first total synthesis of a denudatine alkaloid (lepenine, 9 ) [25] , while Gin et al realized a refined synthesis of the hetisine-type alkaloid nominine ( 10 ) [19] . Very recently, an elegant approach to weisaconitine D ( 11 ) and liljestrandinine ( 12 ) was developed by Sarpong and co-workers employing a network analysis strategy [27] , which has enabled this area to reach new technical heights. Despite these advances, the total synthesis of the unique arcutane/arcutine group (for example, atropurpuran 3 and arcutinine 6 ) has been impeded by the complexity of the cage-like tetracyclo[5.3.3.0 4,9 .0 4,12 ]tridecane unit (blue bonds shown in Fig. 1a ). Aside from the bridged ring systems, the challenging task was further complicated by the presence of multiple stereogenic centres embedded in the molecules, including two all-carbon bridgehead quaternary centres (C5 and C8). These natural products have been the focus of many synthetic studies [29] , [30] , [31] , [32] due not only to their alluring structures, but also because their biological functions are unknown. Here, we describe our recent endeavours that led to the first total synthesis of (±)-atropurpuran. Retrosynthetic analysis Our retrosynthetic analysis is outlined in Fig. 2 . The target molecule atropurpuran ( 3 ) could be accessed through functional group manipulations from an advanced intermediate 13 . Central to the synthesis of 3 would be the assembly of its core structure (that is, 13 ), which can be realized from keto aldehyde 14 via a sequence of aldol addition and ketyl-olefin cyclization [33] . Construction of the C5–C20 bond before the C9–C10 bond would be critical for delivering the right stereochemical outcome at C9. We speculated that the precursor 14 could in turn be obtained by a reductive Knoevenagel condensation [34] between 1,3-cyclohexanedione ( 15 ) and aldehyde 16 . Generation of tricycle 17 (the precursor of 16 ) would rely on an oxidative dearomatization/intramolecular Diels-Alder cycloaddition (IMDA) cascade reaction from the olefinic phenol 18 , which has been proven to be efficient for stereoselective synthesis of bicyclo[2.2.2]octane systems [35] . 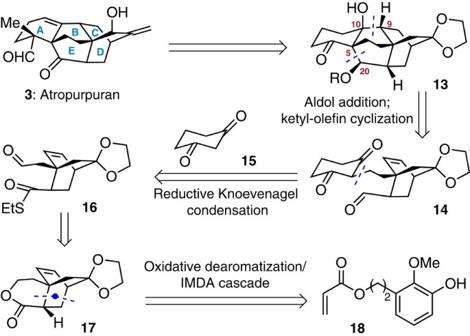Figure 2: Retrosynthetic analysis of atropurpuran (3). The key disconnections involve an aldol reaction and a ketyl-olefin cyclization to construct rings E and B, respectively, at a late stage. Figure 2: Retrosynthetic analysis of atropurpuran (3). The key disconnections involve an aldol reaction and a ketyl-olefin cyclization to construct rings E and B, respectively, at a late stage. Full size image Synthesis of the pentacyclic core structure The multiple step synthesis begins with preparation of the tricyclic intermediate 17 as shown in Fig. 3a . Homologation of readily available aldehyde 19 (ref. 36 ) was achieved using the in situ generated ylide Ph 3 P=CHOMe followed by workup; reduction of the resultant aldehyde gave alcohol 20 in 55% overall yield in two steps. Subjecting 20 to a sequence of esterification with acryloyl chloride and desilylation by TBAF (tetra- n -butylammonium fluoride) generated the olefinic phenol 18 . Having a rapid approach to the precursor 18 established, the stage was thus set for the crucial oxidative dearomatization/IMDA cascade reaction. As anticipated, phenol 18 underwent facile oxidation on exposure to PIDA (iodobenzene diacetate) in MeOH. After switching the solvent from methanol to xylene, the ensuing IMDA cycloaddition proceeded smoothly at 150 °C through the endo transition state ( 21 ), securing the desired bicyclo[2.2.2]octane unit ( 22 ) as a single diastereomer ( Supplementary Figs 11–13 ). Removal of the two methoxy groups in 22 in the presence of SmI 2 (ref. 37 ) followed by subsequent ketone protection furnished 17 in 76% overall yield. 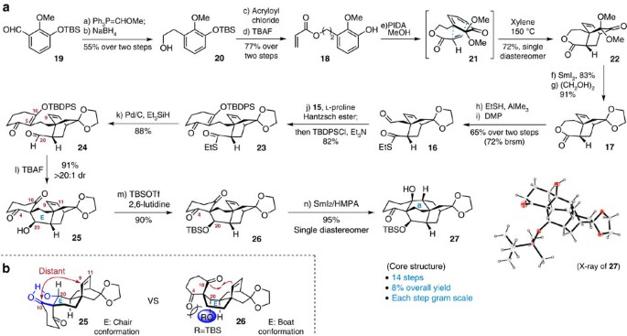Figure 3: Access to the core structure for both arcutane diterpenes and arcutine alkaloids. (a) Conditions: (a) Ph3PCH2OMeCl,t-BuOK, THF, 0 °C; then TMSCl, NaI, MeCN, −18 °C; (b) NaBH4, MeOH, 0 °C, 55% over two steps; (c) acryloyl chloride, Et3N, CH2Cl2, rt; (d) TBAF, THF, rt, 77% over two steps; (e) PIDA, MeOH, 0 °C; then xylene, BHT, 150 °C; 72%; (f) SmI2, THF/MeOH (20:1), rt, 83%; (g) ethylene glycol, TMSCl, CH2Cl2, rt, 91%; (h) EtSH, AlMe3, CH2Cl2, 0 °C to rt; (i) DMP, CH2Cl2, rt, 65% over two steps (72% brsm); (j) 1,3-cyclohexanedione (15), Hantzsch ester,L-proline, CH2Cl2; then TBDPSCl, Et3N, CH2Cl2, rt, 82%; (k) Pd/C, Et3SiH, CH2Cl2, rt, 88%; (l) TBAF, THF, rt, 91% (>20:1 dr); (m) TBSOTf, 2,6-lutidine, CH2Cl2, –40 °C, 90%; (n) SmI2, HMPA, THF/t-BuOH (20:1), rt, 95%. (b) Comparison of the conformational preferences of intermediates25and26. BHT, 2,6-bis(1,1-dimethylethyl)-4-methylphenol; brsm, based on recovered starting material; HMPA, hexamethylphosphoramide; PIDA, iodobenzene diacetate; TBAF, tetra-n-butylammonium fluoride; TBDPSCl,tert-butyl(chloro)diphenylsilane; TBS,tert-butyldimethylsilyl; TBSOTf,tert-butyldimethylsilyl trifluoromethanesulfonate; THF, tetrahydrofuran; TMSCl, chlorotrimethylsilane. Figure 3: Access to the core structure for both arcutane diterpenes and arcutine alkaloids. ( a ) Conditions: (a) Ph 3 PCH 2 OMeCl, t -BuOK, THF, 0 °C; then TMSCl, NaI, MeCN, −18 °C; (b) NaBH 4 , MeOH, 0 °C, 55% over two steps; (c) acryloyl chloride, Et 3 N, CH 2 Cl 2 , rt; (d) TBAF, THF, rt, 77% over two steps; (e) PIDA, MeOH, 0 °C; then xylene, BHT, 150 °C; 72%; (f) SmI 2 , THF/MeOH (20:1), rt, 83%; (g) ethylene glycol, TMSCl, CH 2 Cl 2 , rt, 91%; (h) EtSH, AlMe 3 , CH 2 Cl 2 , 0 °C to rt; (i) DMP, CH 2 Cl 2 , rt, 65% over two steps (72% brsm); (j) 1,3-cyclohexanedione ( 15 ), Hantzsch ester, L -proline, CH 2 Cl 2 ; then TBDPSCl, Et 3 N, CH 2 Cl 2 , rt, 82%; (k) Pd/C, Et 3 SiH, CH 2 Cl 2 , rt, 88%; (l) TBAF, THF, rt, 91% (>20:1 dr); (m) TBSOTf, 2,6-lutidine, CH 2 Cl 2 , –40 °C, 90%; (n) SmI 2 , HMPA, THF/ t -BuOH (20:1), rt, 95%. ( b ) Comparison of the conformational preferences of intermediates 25 and 26 . BHT, 2,6-bis(1,1-dimethylethyl)-4-methylphenol; brsm, based on recovered starting material; HMPA, hexamethylphosphoramide; PIDA, iodobenzene diacetate; TBAF, tetra- n -butylammonium fluoride; TBDPSCl, tert -butyl(chloro)diphenylsilane; TBS, tert -butyldimethylsilyl; TBSOTf, tert -butyldimethylsilyl trifluoromethanesulfonate; THF, tetrahydrofuran; TMSCl, chlorotrimethylsilane. Full size image The next step was to assemble the pentacyclic backbone of atropurpuran ( Fig. 3a ). The cleavage of the lactone in 17 with EtSH, followed by Dess-Martin oxidation of the resultant primary alcohol, led to aldehyde 16 in 65% overall yield. A reductive Knoevenagel condensation between 1,3-cyclohexanedione ( 15 ) and aldehyde 16 took place smoothly utilizing L -proline as the catalyst and Hantzsch ester as the hydrogen source. Given the limited stability of the resulting product, this intermediate was masked immediately as an enol silane in one pot to give thioester 23 in 82% yield. Conversion of thioester 23 into aldehyde 24 was readily achieved according to Fukuyama’s protocol [38] . At this point, we were faced with the construction of two critical C–C bonds (that is, C5–C20 and C9–C10) before arriving at the pentacyclic framework of the target molecule. We reasoned that establishment of the C5–C20 bond first would be beneficial to the installation of the requisite stereocenter at C9. As a result, subjection of the labile silyl enol ether ( 24 ) to TBAF secured the formation of the E ring to afford tetracyclic diketone 25 and its 20-hydroxyl epimer (91% yield, >20:1 dr). With the aforementioned strategy in mind, we then focused on investigating the pivotal ketyl-olefin cyclization to set up the B ring. After much experimentation, the cyclization of 25 proved to be challenging in that the starting material remained under most attempted conditions using SmI 2 as a radical initiator. This could be explained by the assumption that a chair conformation was adopted for the E ring due to its tendency to release the steric repulsion between the cyclohexanedione and the bridged bicyclo[2.2.2]octane system ( 25 , Fig. 3b ), which resulted in a significant spatial distance between the generated ketyl radical at C10 and the radical acceptor of Δ [9] , [11] olefin. In addition, the intramolecular H-bonding between the proximal ketone and free hydroxyl group might stabilize this chair conformation. In this context, we hypothesized that a bulky substituent at the C20 position would not only interrupt the H-bonding but also force the formation of a boat conformation for the E ring because of the steric repulsion between the bulky OR group at C20 and the ketone group at C4 ( 26 , Fig. 3b ). In the boat conformation, the ketone moiety at C10 was in close proximity to the olefin, thus favouring the desired cyclization [33] . Working on this hypothesis, a bulky TBS protecting group was then installed on the C20 hydroxyl group in 25 to give 26 . Gratifyingly, on treatment of intermediate 26 with SmI 2 /HMPA, the expected cyclization proceeded with remarkable efficiency to yield 27 as a single diastereomer in 95% yield. Its structure was unambiguously confirmed by X-ray crystallographic analysis (see Supplementary Methods ). Overall, the 14-step sequence enabled an efficient access to the core structure for both arcutane diterpenes and arcutine alkaloids on a gram scale. Total synthesis of atropurpuran The final steps of our synthesis of (±)-atropurpuran are illustrated in Fig. 4 . Dehydration of the tertiary hydroxyl group in 27 with SOCl 2 in pyridine, followed by removal of dioxolane in aqueous acetone, afforded diketone 28 in 67% overall yield. A three-step transformation including selective Wittig methylenation at C16, Corey-Chaykovsky epoxidation [39] at C4, and epoxide opening with BF 3 ·OEt 2 (ref. 40 ) enabled access to aldehyde 29 as a single diastereomer for further methylation at C4. The stereochemistry of the aldehyde group in 29 was not determined at this stage. Because the initial efforts for α-methylation of aldehyde 29 failed, probably due to its sterically hindered environment, desilylation was conducted using TBAF, leading to a pair of inseparable hydroxyl aldehydes along with corresponding mixtures of a cyclic hemiacetal. On treating the above crude mixture with Dess-Martin periodinane, clean keto aldehyde 30 was obtained as a pair of separable diastereomers ( ∼ 1:1 dr). As anticipated, under the conditions of t -BuOK/MeI, both diastereomers were converted to the desired product 31 and its C4 methyl epimer in 75% yield (5:1 dr) based on recycling of 30a/b ( Supplementary Methods ). 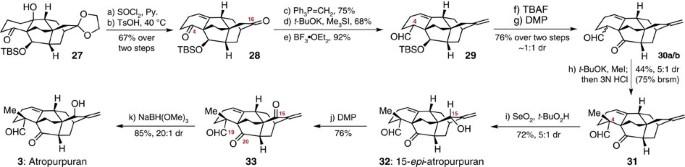Figure 4: Completion of the total synthesis of (±)-atropurpuran (3). Conditions: (a) SOCl2, Py., 0 °C; (b) TsOH, acetone/H2O (10:1), 40 °C, 67% over two steps; (c) Ph3PCH3Br,t-BuOK, PhMe, rt, 75%; (d) Me3SI,t-BuOK, DMSO, THF, rt, 68%; (e) BF3·OEt2, PhMe, –20 °C, 92%; (f) TBAF, THF, reflux; (g) DMP, CH2Cl2, rt, 76% over two steps (∼1:1 dr); (h)t-BuOK, MeI,t-BuOH, rt; then 3N HCl, THF, 44% (75% brsm, 5:1 dr); (i) SeO2,t-BuO2H, CH2Cl2, 30 °C, 72% (5:1 dr); (j) DMP, CH2Cl2, rt, 76%; (k) NaBH(OMe)3, THF/MeOH (10:1), −30 °C, 85% (20:1 dr). DMP, Dess-Martin periodinane; THF, tetrahydrofuran. Figure 4: Completion of the total synthesis of (±)-atropurpuran (3). Conditions: (a) SOCl 2 , Py., 0 °C; (b) TsOH, acetone/H 2 O (10:1), 40 °C, 67% over two steps; (c) Ph 3 PCH 3 Br, t -BuOK, PhMe, rt, 75%; (d) Me 3 SI, t -BuOK, DMSO, THF, rt, 68%; (e) BF 3 ·OEt 2 , PhMe, –20 °C, 92%; (f) TBAF, THF, reflux; (g) DMP, CH 2 Cl 2 , rt, 76% over two steps ( ∼ 1:1 dr); (h) t -BuOK, MeI, t -BuOH, rt; then 3N HCl, THF, 44% (75% brsm, 5:1 dr); (i) SeO 2 , t -BuO 2 H, CH 2 Cl 2 , 30 °C, 72% (5:1 dr); (j) DMP, CH 2 Cl 2 , rt, 76%; (k) NaBH(OMe) 3 , THF/MeOH (10:1), −30 °C, 85% (20:1 dr). DMP, Dess-Martin periodinane; THF, tetrahydrofuran. Full size image With 31 in hand, we envisioned that an allylic oxidation of the exocyclic alkene might give access to our target. However, the oxidation occurred predominately from the less hindered α face and produced the undesired 15-epi-atropurpuran 32 as the major product, along with the minor product atropurpuran 3 . Interestingly, the yield and diastereomeric ratio for the allylic oxidation were observed to be 45% and 14:1, respectively, when using an old SeO 2 stored in our laboratory, while the yield increased to 72% and the dr value dropped to 5:1 with a freshly ordered SeO 2 , possibly owing to the different reactivity of the two reagents (see Supplementary Methods ). After extensive experimentation, inversion of the stereochemistry of the C15 hydroxyl group in 32 proved to be fruitless. In this context, we turned to an oxidation–reduction sequence for setting up the right stereochemistry at C15, which seemed challenging but possible. On one hand, hydride attack to the ketone at C15 ( 33 ) from the less hindered α face during the reduction would stereoselectively generate the desired C15 hydroxyl group. Furthermore, a chemoselective reduction could be realized through a substrate-controlled manner, owing to the crowded circumstances of two carbonyl groups at C19 and C20 compared with that of C15. Thus, enone 33 was readily prepared via Dess-Martin oxidation of alcohol 32 , before we screened the reduction conditions in detail. Initially, reductants such as reactive diisobutylaluminium hydride, lithium tri- sec -butylborohydride ( L -selectride), and NaBH 4 –CeCl 3 resulted in over-reduction even at a low temperature (–78 °C). In contrast, no reaction was observed using the less reactive sodium triacetoxyborohydride, sodium triethylborohydride and potassium tri- sec -butylborohydride (K-selectride) at temperatures below –30 °C. Finally, it was found that reduction of enone 33 with NaBH 4 at –60 °C in tetrahydrofuran/MeOH (10:1) for 1 h provided atropurpuran 3 and 15- epi -atropurpuran 32 in 75% yield and 2:1 dr, without reduction of the carbonyl groups at C19 and C20. The stereoselectivity was greatly improved to 20:1 dr to give atropurpuran 3 with 85% yield when more bulky sodium trimethoxyborohydride was employed as the reductant at –30 °C in tetrahydrofuran/MeOH (10:1) for 16 h. The spectral data of synthetic atropurpuran 3 were identical in all respects to those reported for the natural product [11] . In summary, we have disclosed an expedient and scalable approach to synthesize the core structure for arcutane diterpenes and related alkaloids and achieved the first total synthesis of (±)-atropurpuran. The oxidative dearomatization/IMDA cascade was employed as a key reaction in constructing the bicyclo[2.2.2]octane ring. Sequential aldol and ketyl-olefin cyclizations were used to secure the highly bridged tetracyclo[5.3.3.0 4,9 .0 4,12 ]tridecane unit with excellent stereoselectivity. Of particular note, a chemoselective [41] and stereoselective reduction allowed us to install the requisite allylic hydroxyl group in the target atropurpuran. Having had success with this synthetic approach, our future efforts will focus on pursuit of an asymmetric version, as well as an extension to the total synthesis of corresponding diterpenoid alkaloids. General All reactions that require anhydrous conditions were performed in flame-dried glassware under Ar atmosphere and all reagents were purchased from commercial suppliers. Solvent purification was conducted according to Purification of Laboratory Chemicals [42] . The products were purified by flash column chromatography on silica gel (200–300 meshes). The reactions were monitored by thin layer chromatography. Visualization was accomplished with ultraviolet light, exposure to iodine, staining with an ethanolic solution of phosphomolybdic acid or basic solution of KMnO 4 . 1 H nuclear magnetic resonance (NMR) and 13 C NMR spectra were recorded on Varian INOVA-400/54 and Agilent DD2-600/54 instruments and calibrated by using residual undeuterated chloroform (δ, 1 H NMR=7.260, 13 C NMR=77.00). The following abbreviations were used to explain the multiplicities: br, broad; d, doublet; dt, double triplet; m, multiplet; s, singlet; t, triplet; td, triple doublet; q=quartet and coupling constants ( J ) are reported in Hertz (Hz). Infrared (IR) spectra were recorded on a Perkin Elmer Spectrum Two fourier transform infrared spectrometer. High-resolution mass spectra were recorded on Bruker Apex IV FTMS or Thermo Scientific LTQ Orbitrap XL ESI mass spectrometers. Experimental data For NMR spectra of synthetic intermediates, see Supplementary Figs 1–52 . For the comparisons of 1 H and 13 C NMR spectra of the natural and synthetic atropurpuran, see Supplementary Figs 53–58 . For the comparisons of 1 H and 13 C NMR spectroscopic data of the natural and synthetic atropurpuran, see Supplementary Tables 1 and 2 . For the experimental procedures and spectroscopic and physical data of compounds and the crystallographic data of compound 27 , see Supplementary Methods . Data availability The X-ray crystallographic coordinates for structure 27 reported in this study have been deposited at the Cambridge Crystallographic Data Centre (CCDC) with the accession code CCDC 1435700 ( www.ccdc.cam.ac.uk/data_request/cif ). The authors declare that all other relevant data supporting the findings of this study are available within the article and its Supplementary Information files. How to cite this article: Gong, J. et al . Total synthesis of atropurpuran. Nat. Commun. 7:12183 doi: 10.1038/ncomms12183 (2016).